Optical sinc-shaped Nyquist pulses of exceptional quality Sinc-shaped Nyquist pulses possess a rectangular spectrum, enabling data to be encoded in a minimum spectral bandwidth and satisfying by essence the Nyquist criterion of zero inter-symbol interference (ISI). This property makes them very attractive for communication systems since data transmission rates can be maximized while the bandwidth usage is minimized. However, most of the pulse-shaping methods reported so far have remained rather complex and none has led to ideal sinc pulses. Here a method to produce sinc-shaped Nyquist pulses of very high quality is proposed based on the direct synthesis of a rectangular-shaped and phase-locked frequency comb. The method is highly flexible and can be easily integrated in communication systems, potentially offering a substantial increase in data transmission rates. Further, the high quality and wide tunability of the reported sinc-shaped pulses can also bring benefits to many other fields, such as microwave photonics, light storage and all-optical sampling. In currently deployed optical networks, wavelength division multiplexing (WDM) is used to enhance the carrier capacity of optical fibres. However, since the data rate in optical networks increases by close to 29% per year [1] , new approaches are being developed [2] . The bulk of these approaches consists in increasing the spectral efficiency of optical links. Using multilevel modulation formats and polarization multiplexing, the spectral efficiency can be increased from 0.8 to several bit s −1 Hz −1 (refs 3 , 4 , 5 ). However, such schemes drastically increase the requirements on electrical signal processing and are typically accompanied by higher energy consumption. To keep pace with the growing demand, a data rate of 1 Tbit s −1 per channel together with high spectral efficiency has been envisaged for the next decade [6] . Even with parallelization, these data rates are beyond the limits of current digital signal processing, and the resulting baud rate exceeds the possibilities of current electronic circuits [7] . A possible solution is the combination of several lower-rate channels with high spectral efficiency into a Tbit s −1 ‘superchannel’, which can be routed through the existing optical networks as a single entity [8] . Such an aggregation can be achieved in the frequency or time domain [9] . In orthogonal frequency-division multiplexing (OFDM), a superchannel consisting of a set of subcarriers is generated. Each subcarrier exhibits a sinc-shaped spectrum and can therefore be spaced at the baud rate without inter-channel interference. With OFDM, a data rate of 26 Tbit s −1 and a net spectral efficiency of 5 bit s −1 Hz −1 have been demonstrated [10] . Similarly, for Nyquist transmission, the symbols are carried by Nyquist pulses [11] that overlap in the time domain without ISI. Recently, a 32.5-Tbit s −1 Nyquist WDM transmission with a net spectral efficiency of 6.4 bit s −1 Hz −1 has been shown [12] . Compared with OFDM, Nyquist pulse shaping has several unique advantages as it reduces the receiver complexity [13] , [14] , is less sensitive to fibre nonlinearities [14] , requires much lower receiver bandwidths [15] and leads to lower peak-to-average power ratios [16] . A general expression in the time domain for the amplitude waveform of Nyquist pulses is [17] , [18] : where τ p is the pulse duration between zero crossings and β is known as a roll-off factor [17] , which is in the range 0≤ β ≤1. Among the class of Nyquist pulses [11] , the sinc-shaped pulse is of particular interest owing to its rectangular spectrum [17] and zero roll-off. This allows minimizing the guard band between optical channels. Theoretically, for a sinc-pulse Nyquist transmission, each symbol consists of a time-unlimited sinc-pulse. However, since causality makes it impossible, periodic pulses are typically used in every experimental demonstration of Nyquist pulse transmission [12] , [13] , [14] , [15] , [16] , [17] , [18] , [19] , [20] . Such transmission systems rely on multiplexing and modulation techniques. A possible scheme is shown in Fig. 1 . Nyquist channels can be multiplexed in time domain; this is designated as orthogonal time-division multiplexing (TDM) [18] , [21] , [22] . The generated sequence is split into N channels, which are then delayed and modulated to transport the channel corresponding data. This requires N modulators, with N being the number of branches or the number of time-domain channels. However, compared with a direct modulation, the baud rate of each modulator is N times reduced. This drastically relaxes the requirements on modulators and electronics. In addition, time-domain channels can be multiplexed at different wavelengths; this is designated as Nyquist WDM [8] where pulses can be generated and modulated for each carrier. Since higher-order modulation formats, multiplexing, transmission and demultiplexing of Nyquist pulses have already been shown elsewhere [12] , [13] , [14] , [15] , [16] , [17] , [18] , here the focus is placed on the generation of a sinc-pulse shape as ideal as possible. 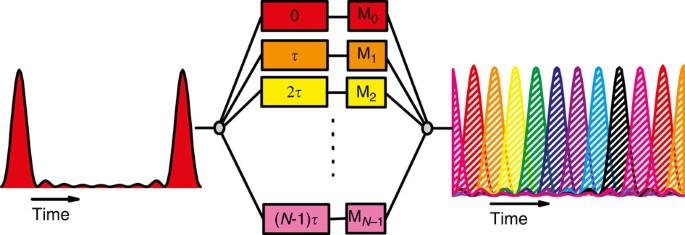Figure 1: Possible multiplexing of sinc-shaped Nyquist pulses. Periodic sinc-pulse sequences can be split intobranches, each of which corresponds to an independent channel. In thenth branch, the periodic sequence is delayed byntimes the intervalτ=1/(NΔf), withn=0,...,N−1. Each channel can be modulated independently with a modulatorM0,...,MN−1. These devices can apply any modulation formats to the signal. Then, theNmodulated channels are multiplexed. The shown multiplexing is carried out in the time domain at one carrier wavelength. Since the multiplexed channel shows a sharp-edged spectrum, the next wavelength channel can be directly adjacent to the previous with almost no guard band and can be multiplexed in the time domain in the same way, reaching high temporal and spectral densities together. Figure 1: Possible multiplexing of sinc-shaped Nyquist pulses. Periodic sinc-pulse sequences can be split into branches, each of which corresponds to an independent channel. In the n th branch, the periodic sequence is delayed by n times the interval τ =1/( N Δ f ), with n =0,..., N −1. Each channel can be modulated independently with a modulator M 0 ,..., M N −1 . These devices can apply any modulation formats to the signal. Then, the N modulated channels are multiplexed. The shown multiplexing is carried out in the time domain at one carrier wavelength. Since the multiplexed channel shows a sharp-edged spectrum, the next wavelength channel can be directly adjacent to the previous with almost no guard band and can be multiplexed in the time domain in the same way, reaching high temporal and spectral densities together. Full size image The temporal and spectral features of sinc-shaped pulses bring benefits not only to optical communications but also to many other fields. Actually, sinc-shaped pulses correspond to the ideal interpolation function for the perfect restoration of band-limited signals from discrete and noisy data [23] . Hence, sinc pulses can provide substantial performance improvement to optical sampling devices [24] . Further, the spectral features of sinc pulses could enable the implementation of ideal rectangular microwave photonics filters [25] , [26] , [27] with tunable passband profiles, thus also providing interesting possibilities for all-optical signal processing [28] , spectroscopy [29] and light storage [30] , [31] . Several approaches for the generation of Nyquist pulses have been suggested. In refs 9 and 16 , an arbitrary waveform generator was programmed offline to create Nyquist filtering of the baseband signal. This can provide a quite good roll-off factor of β =0.0024 (ref. 16 ). However, this method is restricted by the speed of electronics because of the limited sampling rate and limited processor capacities, whereas the quality of the Nyquist pulses highly depends on the resolution (number of bits) of digital-to-analogue converters [32] . Another possibility is the optical generation of Nyquist pulses [13] , [18] , [20] . These optical sequences can reach much shorter time duration and can thus be multiplexed to an ultrahigh symbol rate. To generate Nyquist pulses, a liquid crystal spatial modulator has been used to shape Gaussian pulses from a mode-locked laser into raised-cosine Nyquist pulses. It is also possible to generate Nyquist pulses using fibre optical parametric amplification, pumped by parabolic pulses, and a phase modulator to compensate the pump-induced chirp [20] . However, compared with electrical pulse shaping, optical Nyquist pulse generation produces much higher roll-off factors [33] , such as β =0.5 (refs 13 , 18 ); therefore, multiplexing using this kind of pulses results in a non-optimal use of bandwidth. Further, most of the reported methods use complex and costly equipment. In this paper, a method to generate a sequence of very high-quality Nyquist pulses with an almost ideal rectangular spectrum ( β ~0) is proposed and demonstrated. The method is based on the direct synthesization of a flat phase-locked frequency comb with high suppression of out-of-band components. It is theoretically demonstrated and experimentally confirmed that this comb corresponds to a periodic sequence of time-unlimited sinc pulses. The wide tunability of the method, using a proof-of-concept experiment based on two cascaded Mach–Zehnder modulators (MZM), is demonstrated over 4 frequency decades. Experimental results also verify the remarkable high quality of the generated pulses, exhibiting in all cases zero roll-off, minimum spectral broadening when modulated and <1% deviation with respect to the ideal sinc shape. These pulses simultaneously show a minimum ISI and a maximum spectral efficiency, making them an attractive solution for high-capacity TDM–WDM systems. Basic concepts Considering that owing to physical limitations the ideal sinc pulse with perfect rectangular optical spectrum has not been demonstrated so far, a different approach for sinc-shaped Nyquist pulse generation is proposed in this paper. The technique is a straightforward way to realize sinc-shaped Nyquist pulses in the optical domain, overcoming the limitations imposed by the speed of electronics. The principle of the method is based on the time–frequency duality described by Fourier analysis, as shown in Fig. 2 . It is well-known that a sinc pulse can be represented by a rectangular spectrum in the Fourier domain (see upper figures in Fig. 2 ), while the frequency content of a train of sinc pulses corresponds to a flat comb with equally spaced components within the bandwidth defined by the single-pulse spectrum (see lower figures in Fig. 2 ). Therefore, instead of shaping a single-sinc pulse, the approach proposed here produces a sequence of sinc pulses directly from the generation of an optical frequency comb having uniformly spaced components with narrow linewidth, equal amplitude and linear-locked phase, together with strong outer-band suppression [34] . As demonstrated in this paper, the pulse sequence obtained from this rectangular frequency comb is strictly identical to the summation of individual time-unlimited sinc pulses, and intrinsically satisfies the zero-ISI Nyquist criterion, similar to the ideal single sinc-shaped pulse. As described in Fig. 2 , the frequency spacing Δ f between adjacent spectral lines determines the pulse repetition period T =1/Δ f , and the rectangular bandwidth N Δ f ( N being the number of lines) defines the zero-crossing pulse duration τ p =2/( N Δ f ). Thus, pulse width and repetition rate can be changed by simply tuning the frequency comb parameters. This feature offers a highly flexible and simple way to adjust the bit rate and bandwidth allocation in an optical network according to actual requirements [35] , [36] , or to change the parameters of optical sampling devices [24] whenever required. 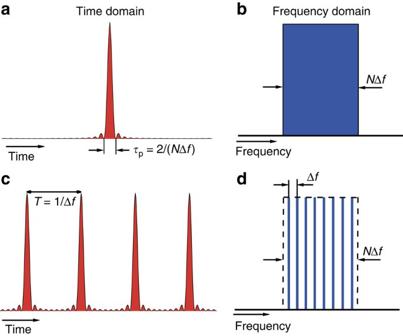Figure 2: Time–frequency correspondence for sinc-shaped Nyquist pulses. Time (left) and frequency (right) representation of a single-sinc pulse (top) and a sinc-pulse sequence (bottom). Since the directly observed quantity in the optical domain is proportional to the optical intensity (or power), here the figure shows the intensity of the time-domain traces instead of the field amplitude. The Fourier domain representation of a sinc pulse (a) is a rectangular function (b), while the spectrum of an unlimited sinc-pulse sequence (c) is a frequency comb with uniform phase under a rectangular envelope (d). Figure 2: Time–frequency correspondence for sinc-shaped Nyquist pulses. Time (left) and frequency (right) representation of a single-sinc pulse (top) and a sinc-pulse sequence (bottom). Since the directly observed quantity in the optical domain is proportional to the optical intensity (or power), here the figure shows the intensity of the time-domain traces instead of the field amplitude. The Fourier domain representation of a sinc pulse ( a ) is a rectangular function ( b ), while the spectrum of an unlimited sinc-pulse sequence ( c ) is a frequency comb with uniform phase under a rectangular envelope ( d ). Full size image Theory The Nyquist criterion for a pulse y ( t ) satisfying zero ISI implies that, for a particular sampling period τ = τ p /2, y ( nτ ) is 0 for any non-zero integer n , while y (0)≠0. This means that when the signal is periodically sampled with a period τ , a non-zero value is obtained only at the time origin [11] . For instance, the sinc function defined as is a Nyquist pulse possessing a rectangular spectrum and is therefore unlimited in time. As a consequence of causality, the sinc function is therefore only a theoretical construct [17] . In this paper, instead of generating a single time-unlimited sinc pulse, a method to obtain a sequence of sinc pulses is proposed based on the generation of a flat frequency comb with close-to-ideal rectangular spectrum. Here it is shown that the time-domain representation of the generated comb corresponds to an unlimited ISI-free summation of sinc-shaped Nyquist pulses. However, in complete contrast to the single-sinc pulse, the pulse sequence can be easily generated from a rectangular frequency comb. Here the mathematical demonstration is presented for an odd number of frequency lines; however, the derivation for an even number can be straightforwardly obtained following the same procedure. The time-domain representation of the optical field of a frequency comb with N lines, having the same amplitude E 0 / N and frequency spacing Δ f around the central frequency f 0 , can be expressed as: For the sake of simplicity, it is assumed that all frequency components have the same phase φ . Strictly speaking, it is sufficient that the phases of all frequency components are locked showing a linear dependence on frequency; however, this linear dependence can be nullified by properly choosing the time origin without the loss of generality. Equal phases will be assumed hereafter to simplify the notation. From equation (2), the normalized envelope of the optical field is calculated to be , denominated hereafter as periodic sinc function. To demonstrate that this envelope actually corresponds to a train of sinc-shaped Nyquist pulses, it is convenient to start from its frequency domain representation. According to equation (2) and using the Fourier transform, it follows: Introducing the rectangular function П that is 1 for all integers n where and 0 elsewhere, the above equation can be written as: where the rectangular spectrum , covering a bandwidth N Δ f , is represented in the time domain by the sinc-pulse N Δ f sinc( N Δ ft ). The temporal dependence of the above expression can then be obtained by taking its inverse Fourier transform and using the Poisson summation formula [37] : where ⊗ denotes the convolution operation. Thus, it follows for the right-hand side of equation (5): Therefore, it can be written that Similarly, for an even number of spectral lines, the envelope of the optical field can be expressed as a train of sinc pulses through the following equation: where the factor (−1) n comes from the absence of a spectral line at the central frequency of the comb; this eliminates the direct current (DC) component in the optical field envelope. Comparing equations (7) and (8), the following general expression for the normalized envelope of the optical field resulting from a flat frequency comb is obtained, independent of the parity of N : The difference in the periodic sinc function for even and odd N can be figured out easily. As depicted in Fig. 3a , all sinc pulses of the pulse train for odd N show the same phase, so that x ( t s )=1 at every sampling instant for all integer n . For even N , x ( t s )=(−1) n , so that each pulse envelope is of opposite sign with its preceding and following pulses, as shown in Fig. 3b . 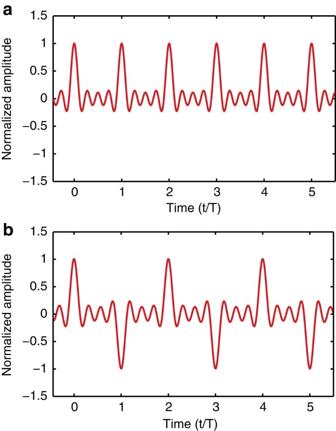Figure 3: Normalized field envelope of a frequency comb. (a) Odd (N=9) and (b) even (N=8) number of spectral lines. The time axis is normalized with respect to the pulse periodT. An odd number of lines leads to a sequence of in-phase sinc-shaped Nyquist pulses, while an even numberNresults in a sequence with alternatedπ-phase-modulated pulses. Aside from this difference, the optical intensity measured by a photodetector is the same in both cases, and is given by: Figure 3: Normalized field envelope of a frequency comb. ( a ) Odd ( N =9) and ( b ) even ( N =8) number of spectral lines. The time axis is normalized with respect to the pulse period T . An odd number of lines leads to a sequence of in-phase sinc-shaped Nyquist pulses, while an even number N results in a sequence with alternated π -phase-modulated pulses. Full size image Consequently, it is proven that the field envelope of the time-domain representation of a frequency comb of N identical and equally spaced lines corresponds to an infinite summation of sinc-shaped Nyquist pulses with period and zero-crossing pulse width . Thus, considering that the pulse repetition period is a multiple of the time interval , the resulting time-domain envelope x(t) satisfies the following condition for any integer m : Thus, the sequence of sinc pulses resulting from a locked phase, rectangular frequency comb satisfies the Nyquist criterion for free ISI within every pulse repetition period T . This condition is automatically and intrinsically satisfied for any flat frequency comb since the number of lines N is an integer by definition. Therefore, the generated sinc-pulse sequence can be multiplexed in time without ISI. Proof-of-concept experiment There are several different approaches for the generation of a frequency comb. For instance, they can be obtained from conventional femtosecond lasers, such as Er-fibre [38] , [39] , Yb-fibre [40] and Ti:sapphire [41] mode-locked lasers, or from a continuous wave optical source exploiting Kerr-nonlinearities in an optical resonator [42] , [43] , [44] , [45] , or employing a combination of strong intensity and phase modulation [46] , [47] , [48] together with chirped Bragg gratings [49] , dispersive medium [50] or highly nonlinear fibres [51] , [52] , [53] . However, every comb does not necessarily result in a sequence of Nyquist pulses, since a sinc-pulse sequence can only be obtained under specific conditions, requiring that the produced comb has to show line amplitudes as equal as possible, linear phase dependence through all lines and a strong suppression of out-of-band lines. Thus, although flat frequency combs can be obtained using different methods, as for instance through phase modulation [48] , [49] , [50] , the phase difference between lines and the existing out-of-band components make phase modulators improper for clean generation of sinc-shaped pulses. In general, a close-to-ideal rectangular-shaped optical frequency comb can be produced using various implementations; for instance, a non-optimal frequency comb [38] , [39] , [40] , [41] , [42] , [43] , [44] , [45] , [46] , [47] , [48] , [49] , [50] , [51] , [52] , [53] can be used in combination with a spectral line-by-line manipulation of the optical Fourier components [54] , [55] to control the amplitude and phase of each spectral line. It turns out that the complexity of this kind of pulse shapers significantly increases with the number of spectral lines, and in general pulse shapers are unable to manipulate a frequency comb having spectrally spaced lines below 1 GHz [54] , [55] . Here a simple proof-of-concept experimental set-up, shown in Fig. 4a , is proposed. This uses two cascaded lithium niobate MZM with a specific adjustment of the bias and modulation voltages (see Methods for details). An optical spectrum analyzer (OSA) with a spectral resolution of 0.01 nm is used to measure the generated frequency combs, while an optical sampling oscilloscope with 500 GHz bandwidth is employed to measure the time-domain pulse train waveforms. While the first modulator, driven by a radio-frequency (RF) signal at a frequency f 1 is adjusted to generate three seeding spectral components, the second MZM re-modulates those lines using an RF signal at f 2 . Thus, for instance, to generate N =9 spectral lines, the condition f 1 =3 f 2 or f 2 =3 f 1 has to be satisfied without any carrier suppression, resulting in a frequency spacing between the lines of Δ f =min( f 1 , f 2 ). However, to generate a comb with N =6 lines, the carrier of one of the modulators must be suppressed leading to two possible configurations, as illustrated in Fig. 4b,c . If the optical carrier is suppressed in the first modulator (see Fig. 4b ), the RF frequencies must satisfy the condition 2 f 1 =3 f 2 , giving a line spacing Δ f = f 2 . On the other hand, if the carrier is suppressed in the second modulator (see Fig. 4c ), the relation between modulating frequencies has to be f 1 =4 f 2 , resulting in a frequency spacing Δ f =2 f 2 . 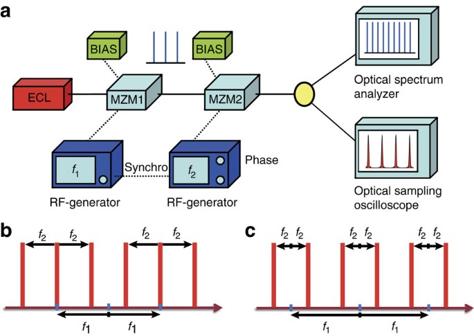Figure 4: Basic experimental implementation. (a) Proof-of-concept set-up. Solid and dashed lines describe optical and electrical connections, respectively. An external cavity laser (ECL) generates a narrow linewidth continuous wave light at 1,550 nm. MZM1 generates spectral lines separated by a frequencyf1. Then, MZM2 re-modulates these seeding components with a frequencyf2. RF power and DC bias in both MZMs are adjusted so that all lines result with the same amplitude and phase, and additional sidebands are highly suppressed. An undistorted waveform is only obtained with a proper adjustment of the relative modulating phase, and therefore both RF generators have been synchronized using a common time base. (b) Generation of a frequency comb withN=6 lines. MZM1 is driven with a frequencyf1and operates in carrier suppression mode, so that MZM2 re-modulates the two seeding lines, with no carrier suppression, at a frequencyf2=Δf. (c) Second option to generate a comb withN=6 spectral lines; in this case, MZM1 is driven with a frequencyf1(no carrier suppression), while MZM2 re-modulates the three seeding components, in carrier suppression mode, at a frequencyf2=f1/4=Δf/2. Figure 4: Basic experimental implementation. ( a ) Proof-of-concept set-up. Solid and dashed lines describe optical and electrical connections, respectively. An external cavity laser (ECL) generates a narrow linewidth continuous wave light at 1,550 nm. MZM1 generates spectral lines separated by a frequency f 1 . Then, MZM2 re-modulates these seeding components with a frequency f 2 . RF power and DC bias in both MZMs are adjusted so that all lines result with the same amplitude and phase, and additional sidebands are highly suppressed. An undistorted waveform is only obtained with a proper adjustment of the relative modulating phase, and therefore both RF generators have been synchronized using a common time base. ( b ) Generation of a frequency comb with N =6 lines. MZM1 is driven with a frequency f 1 and operates in carrier suppression mode, so that MZM2 re-modulates the two seeding lines, with no carrier suppression, at a frequency f 2 =Δ f . ( c ) Second option to generate a comb with N =6 spectral lines; in this case, MZM1 is driven with a frequency f 1 (no carrier suppression), while MZM2 re-modulates the three seeding components, in carrier suppression mode, at a frequency f 2 = f 1 /4=Δ f /2. Full size image A high-quality rectangular-shaped frequency comb can be obtained by tuning the DC bias V B and the RF voltage amplitude ν s of each modulator following the description presented in the Methods section. To ensure that the three components generated by each modulator are in phase, V B and ν s might take either positive or negative values. Moreover, to obtain spectral lines with similar phase using two cascaded MZMs, the phase difference between the modulating RF signals has to be finely adjusted to compensate propagation delays in optical and electrical links, thus leading to almost perfectly shaped symmetric pulses. On the other hand, to confine the sinc-pulse sequence into the Nyquist bandwidth, a low modulating voltage ν s must be used to strongly suppress the out-of-band components. In particular, the RF-driving voltage ν s of both modulators is here adjusted to remain below ~0.36 V π (where V π is the half-wave voltage of the MZM), securing a suppression of more than 27 dB for the out-of-band components. Note that this level of confinement is only possible, thanks to the two degrees of freedom provided by intensity modulators, since both operating bias point and modulating voltages can be adjusted. Quality and tunability of the sinc-shaped Nyquist pulses The quality of the pulses and the flexibility of the method have been experimentally verified by changing the modulating signal frequencies f 1 and f 2 in a wide spectral range, and comparing measurements with the theoretical expectations. This way different frequency combs with N =9 spectral components have been generated with a frequency spacing Δ f spanning over many decades (between 10 MHz and 10 GHz). In Fig. 5 , the measured sinc pulses (black straight lines) are compared with the theoretical ones (red-dashed lines) described by equation (10). Measured and theoretical curves are normalized in all figures. Temporal waveforms have been acquired with a sampling interval of 0.2 ps for the case of Δ f =10 GHz; this interval has been proportionally increased for longer pulse widths. In particular, Fig. 5a shows the case of modulating frequencies f 1 =30 MHz and f 2 =Δ f =10 MHz, resulting in sinc-shaped Nyquist pulses with zero-crossing pulse duration of τ p =22.22 ns, full-width at half-maximum (FWHM) duration of 9.8 ns and a repetition period of T =100 ns. In Fig. 5b–d , the modulating frequencies have been sequentially increased by one order of magnitude. It is observed that the generated pulse sequences coincide very well with the ideal ones over 4 frequency decades, showing a root mean square (r.m.s.) error below 1% for all cases. In addition, it was verified that the spectrum for all these conditions resulted to be close to the ideal rectangular case, as it will be detailed below. 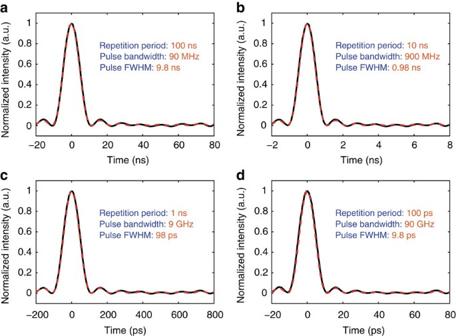Figure 5: Tunability of sinc-shaped Nyquist pulses using nine spectral lines. Sinc-shaped Nyquist pulses measured using a 500-GHz optical sampling oscilloscope. The calculated waveforms (red-dashed lines) according to equation (10) are compared with the measured pulses (black straight lines) for different bandwidth conditions over 4 decades. Nyquist pulses are obtained from the generation of a rectangular frequency comb with nine phase-locked components spanning over a spectral width between 90 MHz and 90 GHz, using modulating frequencies (a)f1=30 MHz andf2=Δf=10 MHz, (b)f1=300 MHz andf2=Δf=100 MHz, (c)f1=3 GHz andf2=Δf=1 GHz, and (d)f1=30 GHz andf2=Δf=10 GHz. The maximum difference between measured pulses and theoretical ones remained in all cases below 1%. Figure 5: Tunability of sinc-shaped Nyquist pulses using nine spectral lines. Sinc-shaped Nyquist pulses measured using a 500-GHz optical sampling oscilloscope. The calculated waveforms (red-dashed lines) according to equation (10) are compared with the measured pulses (black straight lines) for different bandwidth conditions over 4 decades. Nyquist pulses are obtained from the generation of a rectangular frequency comb with nine phase-locked components spanning over a spectral width between 90 MHz and 90 GHz, using modulating frequencies ( a ) f 1 =30 MHz and f 2 =Δ f =10 MHz, ( b ) f 1 =300 MHz and f 2 =Δ f =100 MHz, ( c ) f 1 =3 GHz and f 2 =Δ f =1 GHz, and ( d ) f 1 =30 GHz and f 2 =Δ f =10 GHz. The maximum difference between measured pulses and theoretical ones remained in all cases below 1%. Full size image The shaded box in Fig. 6a shows an ideal rectangular spectrum, which corresponds to a single-sinc pulse with a FWHM duration of 9.8 ps, as the one reported in Fig. 5d . The red curve represents the measured flat phase-locked comb in such a case, showing more than 27 dB suppression of the higher-order sidebands and a power difference between components lower than 0.2 dB. The pulse repetition period, corresponding to T =100 ps, is clearly observed in Fig. 6b . 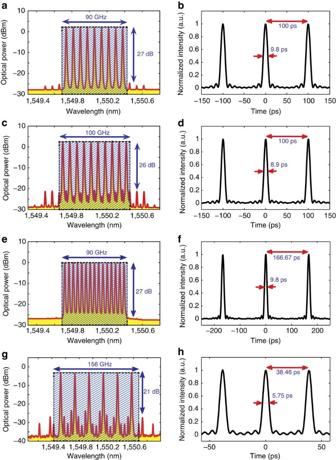Figure 6: Frequency and time-domain representation of the generated sinc-shaped Nyquist pulses. Pulse duration and repetition rate can be easily modified by adjusting the bias voltage of the modulators as well as the frequency and amplitude of modulating signals. Frequency combs with different bandwidth and number of spectral components have been experimentally generated. (a) Measured spectrum and (b) measured time-domain waveform of a comb generated withN=9 spectral components separated by Δf=10 GHz, and expanding over a bandwidth of 90 GHz. (c) Spectrum and (d) time-domain waveform of a comb generated withN=10, Δf=10 GHz, and bandwidth of 100 GHz. (e) Spectrum and (f) time-domain waveform of a comb generated withN=15, Δf=6 GHz, and bandwidth of 90 GHz. (g) Spectrum and (h) time-domain waveform of a comb withN=6, Δf=26 GHz, and an extended bandwidth of 156 GHz. The comb has been spectrally broadened using the second-order sidebands of the first MZM. A power difference among spectral components lower than 0.2 dB is obtained in all cases. The shaded boxes ina,c,eandgrepresent the theoretical Nyquist bandwidth of the generated sinc pulses. Spectral measurements are obtained with a resolution of 0.01 nm, temporal waveforms acquired with a 500-GHz optical oscilloscope using a sampling interval of 0.2 ps and two time-averaged traces. Only the waveform inhis measured with eight times averaging. Figure 6: Frequency and time-domain representation of the generated sinc-shaped Nyquist pulses. Pulse duration and repetition rate can be easily modified by adjusting the bias voltage of the modulators as well as the frequency and amplitude of modulating signals. Frequency combs with different bandwidth and number of spectral components have been experimentally generated. ( a ) Measured spectrum and ( b ) measured time-domain waveform of a comb generated with N =9 spectral components separated by Δ f =10 GHz, and expanding over a bandwidth of 90 GHz. ( c ) Spectrum and ( d ) time-domain waveform of a comb generated with N =10, Δ f =10 GHz, and bandwidth of 100 GHz. ( e ) Spectrum and ( f ) time-domain waveform of a comb generated with N =15, Δ f =6 GHz, and bandwidth of 90 GHz. ( g ) Spectrum and ( h ) time-domain waveform of a comb with N =6, Δ f =26 GHz, and an extended bandwidth of 156 GHz. The comb has been spectrally broadened using the second-order sidebands of the first MZM. A power difference among spectral components lower than 0.2 dB is obtained in all cases. The shaded boxes in a , c , e and g represent the theoretical Nyquist bandwidth of the generated sinc pulses. Spectral measurements are obtained with a resolution of 0.01 nm, temporal waveforms acquired with a 500-GHz optical oscilloscope using a sampling interval of 0.2 ps and two time-averaged traces. Only the waveform in h is measured with eight times averaging. Full size image Then, the pulse duration and the repetition rate have been easily changed by modifying the spectral characteristics of the generated frequency comb. For instance, if the second modulator is driven by two RF signals combined in the electrical domain, each of the three frequency components resulting from the first MZM are modulated to create up to five spectral lines each (four sidebands and carrier). This way, N =10 spectral lines separated by Δ f =10 GHz have been generated by modulating the first MZM at f 1 =25 GHz in carrier suppression mode and by driving the second MZM with two RF signals at f 21 =10 GHz and f 22 =20 GHz. The measured optical spectrum, showing a bandwidth of 100 GHz and spurious components suppressed by more than 26 dB, is illustrated in Fig. 6c . Note that in this case, the first modulator is working in carrier suppression mode and, therefore, the main spurious lines observed in the spectrum result predominantly from the limited extinction ratio of the modulators (in this case, 40 GHz MZMs with typical extinction ratio of about 23–25 dB), which makes a perfect carrier suppression impossible. Higher suppression of such spurious components can be obtained using modulators with better extinction ratio (note that MZMs with 40 dB extinction ratio are commercially available at 10 GHz bandwidth). Since the frequency spacing among components is the same as in the previous case, that is, Δ f =10 GHz, the pulse repetition period T =100 ps has not changed; however, the zero-crossing pulse duration has been reduced down to τ p =20 ps (FWHM duration of 8.9 ps), as shown in Fig. 6d . By rearranging the modulating frequencies to f 1 =30, f 21 =6 and f 22 =12 GHz, and by adjusting the bias point of the first modulator (see equation (14) in the Methods), so that the carrier is not suppressed in this case, a frequency comb expanding over a bandwidth of 90 GHz has been obtained, with N =15 spectral components, a frequency spacing Δ f =6 GHz and more than 27 dB suppression of higher-order sidebands, as reported in Fig. 6e . The measured sinc pulse has a zero-crossing duration of τ p =22 ps (FWHM duration of 9.8 ps) and a repetition period of T =166.67 ps, as depicted in Fig. 6f . Finally, the bandwidth of the comb has been broadened exploiting the second-order sidebands of the modulators. As described in the Method section, this can be achieved by using a proper DC bias voltage that suppresses simultaneously all odd-order sidebands; but it also requires a modulating amplitude of ν s ≈1.52 V π for a complete carrier suppression. For the MZMs used here, this optimal modulating amplitude corresponds to an RF power of about 1 W. Using standard drivers, it was not possible to reach such an RF power level and suppress completely the carrier, although a strong suppression of unwanted sidebands could be reached by a simple DC bias adjustment. As a workaround, two narrowband fibre Bragg gratings (3 GHz bandwidth each), centred at the carrier wavelength, have been placed at the output of the first MZM, providing more than 40 dB carrier rejection (an optical isolator has also been inserted between the fibre Bragg gratings to avoid multiple reflexions). Thus, driving the first MZM at f 1 =19.5 GHz, two frequency components (second-order sidebands) are obtained with a spectral separation of 78 GHz. Then, the second MZM is driven at f 2 =26 GHz to obtain a comb expanding over a bandwidth of 156 GHz, with N =6 spectral components equally spaced by Δ f =26 GHz. The obtained comb is shown in Fig. 6g , presenting a 21-dB suppression of unwanted components. In the time domain, the measured sinc pulse has a zero-crossing duration of τ p =12.8 ps (FWHM duration of 5.75 ps) and a repetition period of T =38.46 ps, as shown in Fig. 6h . Note that the apparent line broadening shown for all frequency components in Fig. 6 results from the limited resolution of the OSA, which is 0.01 nm. The real linewidth is essentially given by the laser linewidth, which is in the kHz range for the used external cavity laser, that is, more than seven orders of magnitude lower than the pulse rectangular bandwidth. 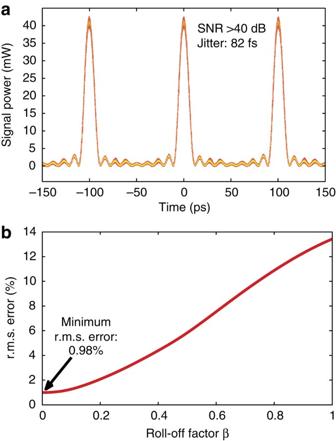Figure 7: High stability and quality of periodic sinc pulses. (a) Colour-grade figure for one of the measured sinc-pulse sequences. In this case, a frequency comb withN=9 spectral components separated by Δf=10 GHz is generated (corresponding to the case depicted inFig. 6a,b, but with no averaging). Measurement indicates a jitter of 82 fs and a SNR>40 dB. Other generated pulse sequences exhibit it similar levels of jitter and SNR. (b) r.m.s. error between measured pulses and the theoretical Nyquist pulse intensity derived from equation (1) as a function of the roll-off factorβ. The r.m.s. error is minimized forβ=0, indicating that the generated pulses match very well the ideal sinc shape with an error of 0.98%. Waveforms measured with other modulating frequencies exhibit similar behaviour. Figure 7a shows a colour-grade plot of the measured Nyquist pulses for the case reported in Fig. 6a,b , demonstrating that even the simple set-up proposed in Fig. 4 can generate very stable and high-quality sinc-shaped pulse sequences with very low jitter (82 fs, equivalent to 0.82% of the FWHM) and very high signal-to-noise ratio (SNR>40 dB, above the oscilloscope SNR measurement capacity). Jitter and SNR for all other measured conditions exhibit similar values with respect to the ones reported here. The quality of the measured pulses is also analyzed by comparing them with the intensity derived from the analytical expression for Nyquist pulses as a function of the roll-off factor β , as described in equation (1). Figure 7b shows the r.m.s. error between the measured pulses and the theoretical intensity waveforms for roll-off factors between 0 and 1. It can be observed that the minimum r.m.s. error is reached with a factor β =0, indicating that the obtained pulses coincide very well with the ideal sinc-pulse shape with an r.m.s. error of 0.98%. All other measurements reported in Figs 5 and 6 also present the same quality as the one described here. When this factor β =0 is compared with the roll-off obtained by other optical pulse-shaping methods [13] , [18] , [20] , [21] (reporting β =0.4 in the best case [21] ), a significant improvement in the quality of the pulses generated here can be easily concluded. This is also evident by simply comparing the spectral and time-domain measurements shown in Figs 5 and 6 with results reported in refs 13 , 18 , 20 and 21 . Figure 7: High stability and quality of periodic sinc pulses. ( a ) Colour-grade figure for one of the measured sinc-pulse sequences. In this case, a frequency comb with N =9 spectral components separated by Δ f =10 GHz is generated (corresponding to the case depicted in Fig. 6a,b , but with no averaging). Measurement indicates a jitter of 82 fs and a SNR>40 dB. Other generated pulse sequences exhibit it similar levels of jitter and SNR. ( b ) r.m.s. error between measured pulses and the theoretical Nyquist pulse intensity derived from equation (1) as a function of the roll-off factor β . The r.m.s. error is minimized for β =0, indicating that the generated pulses match very well the ideal sinc shape with an error of 0.98%. Waveforms measured with other modulating frequencies exhibit similar behaviour. Full size image In conclusion, a simple technique to produce sinc-shaped Nyquist pulses of unprecedented high quality has been proposed and demonstrated based on the optical generation of a phase-locked frequency comb with a rectangular spectral shape. The method offers a high flexibility to modify the pulse parameters, thanks to the possibility of easily changing the bandwidth of the comb, the number of spectral lines and their frequency separation. Because of its conceptual simplicity, many experimental variants can be implemented using similar approaches. In the context of telecommunication systems, the generated sequence of sinc-shaped pulses can be multiplexed either in the time or frequency domain following the standard approaches for orthogonal TDM [18] or Nyquist WDM [8] transmission schemes. To implement an almost ideal Nyquist transmission system, the zero-ISI criterion has to be satisfied by the modulated channels as well. However, it is important to mention that the nearly ideal rectangular spectra reported in Fig. 6 will no longer be obtained if pulses are modulated with data. Since a modulation in time domain corresponds to a convolution in the frequency domain, the spectrum of the modulated sinc-shaped pulses is given by the convolution of the frequency comb and the frequency representation of the modulating signal. Assuming an ideal rectangular modulation window equal to the pulse repetition period T =1/Δ f , the frequency comb will be convolved with a sinc function in the frequency domain [9] having zero crossings at n ·1/ T = n ·Δ f , with n being a non-zero integer number. Thus, the frequency components of the comb coincide with the zero crossings of the modulating signal, which also holds for neighbouring WDM channels (assuming zero guard band). 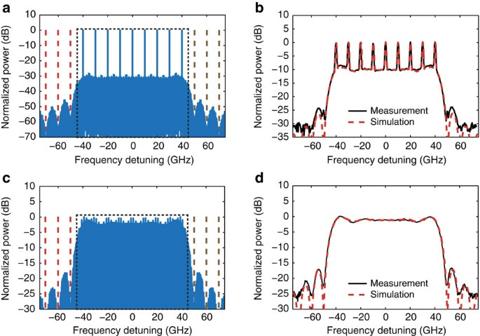Figure 8: Spectrum of modulated sinc pulses. (a) Simulated spectrum resulting from modulating ideal sinc-shaped pulses with on-off keying (OOK) format, using an ideal rectangular modulating window. (b) Measured spectrum obtained from the OOK modulation of the generated sequence of sinc-shaped pulses using a pseudo-random binary sequence of length 231−1. The measured spectrum (black straight line) is compared with the simulated one reported inaconvolved with the finite spectral bandwidth (0.01 nm) of the OSA (red-dashed line). (c) Simulated spectrum resulting from modulating ideal sinc-shaped pulses with binary phase-shift keying (BPSK) format using an ideal rectangular modulating window. (d) Measured spectrum obtained from modulating the generated sequence of sinc-shaped pulses with BPSK. The measured spectrum (black straight line) is compared with the simulated one reported incconvolved with the filtering bandwidth of the OSA (red-dashed line). The dotted boxes inaandcshow the rectangular spectrum of one single pulse and the dashed lines indicate the position of the two adjacent WDM channels, showing that although the spectrum is broadened by the modulation, no guard band between the channels is necessary. Figure 8a and c shows the simulated spectra resulting from modulating ideal sinc pulses with on-off keying and binary phase-shift keying modulation formats, respectively. It is possible to observe the expected spectral broadening resulting from the modulation. As can be seen from the dashed lines, the spectral zero crossings outside the Nyquist bandwidth fall exactly in the comb lines of the adjacent WDM channels, indicating that no guard band between the channels is necessary. Thus, this results in an optimal exploitation of the bandwidth. Both simulated conditions have been experimentally verified by modulating the generated sequence of sinc-shaped pulses using a pseudo-random binary sequence with a length of 2 31 –1. Figure 8b and d compares the spectral measurements (for on-off keying and binary phase-shift keying modulation, respectively) with the spectrum resulting from the simulations convolved with the spectral response of the OSA (a resolution filter with 0.01 nm bandwidth). It is clearly observed that when the generated sinc pulses are modulated, the spectral broadening matches very well the expected behaviour described by the simulations. The small differences between simulation and experiment come from the non-ideal rectangular modulation window and additional convolutions between the very small out-of-band comb lines and the modulation spectrum. Figure 8: Spectrum of modulated sinc pulses. ( a ) Simulated spectrum resulting from modulating ideal sinc-shaped pulses with on-off keying (OOK) format, using an ideal rectangular modulating window. ( b ) Measured spectrum obtained from the OOK modulation of the generated sequence of sinc-shaped pulses using a pseudo-random binary sequence of length 2 31 −1. The measured spectrum (black straight line) is compared with the simulated one reported in a convolved with the finite spectral bandwidth (0.01 nm) of the OSA (red-dashed line). ( c ) Simulated spectrum resulting from modulating ideal sinc-shaped pulses with binary phase-shift keying (BPSK) format using an ideal rectangular modulating window. ( d ) Measured spectrum obtained from modulating the generated sequence of sinc-shaped pulses with BPSK. The measured spectrum (black straight line) is compared with the simulated one reported in c convolved with the filtering bandwidth of the OSA (red-dashed line). The dotted boxes in a and c show the rectangular spectrum of one single pulse and the dashed lines indicate the position of the two adjacent WDM channels, showing that although the spectrum is broadened by the modulation, no guard band between the channels is necessary. Full size image Measurements and simulations indicate that a spectral broadening, so-called excess bandwidth [17] , of about 11% results from modulating the generated sinc pulses (considering only the power within the main spectral lobe, confining about 99% of the power). However, different from other optical pulse-shaping techniques [13] , [18] , [21] , it is important to notice that this excess bandwidth, expressed as a percentage of the Nyquist frequency, does not depend on the roll-off factor of the unmodulated pulses, since this factor is practically zero in the present case. Instead, the broadening here is only given by the ratio between the pulse repetition rate (defining the modulating window) and the pulse width (defining the Nyquist bandwidth) [9] , [17] , thus being proportional to Δ f /( N Δ f )=1/ N (where N is the number of lines in the comb). It is therefore remarkable that even with only N =9 spectral lines, the excess bandwidth resulting from modulation, equal to 1/ N =0.11 and here obtained with a simple proof-of-concept set-up, is significantly lower than the one obtained by other optical pulse-shaping methods [13] , [18] , [21] . Such methods actually report a roll-off factor between β =0.4 (ref. 21 ) and β =0.5 (refs 13 , 18 ) for unmodulated pulses, which is already higher than the factor 0.11 obtained here after modulation. In addition, because of the fixed relation between the symbol duration of the modulating data and the pulse width, this broadening does not require a guard band between WDM channels, as already discussed. It is worth mentioning that the spectral broadening obtained here can be significantly reduced if the number of lines in the frequency comb is increased [9] , [32] . This results in an extension of the modulating window (that is, a narrower modulating spectrum) and/or in a broadening of the Nyquist bandwidth. Thus, for instance, if the pulses in Fig. 6f are modulated, the excess bandwidth would be reduced down to 6.7%. This way, and because of the zero roll-off of the unmodulated pulses, the spectrum of the modulated periodic sinc pulses can expectedly get closer to an ideal rectangular shape [9] , [32] . Finally, in a more general context, it is expected that the use of nearly ideal optical sinc-shaped pulses would not only increase the transmission data rates in existing optical networks but can also provide great benefits for optical spectroscopy, all-optical sampling devices and photonic analogue-to-digital converters, among other potential applications. Rectangular-shaped frequency comb generation Consider M intensity modulators, so that each of them can generate two or three equal-intensity, phase-locked main spectral lines by controlling its DC bias voltage and RF signal amplitude. The impact of the higher-order sidebands will be addressed in a second stage. If a subset of m modulators each creates three spectral lines (carrier and two first-order sidebands) and the remaining M − m modulators each produces two lines (two first-order sidebands with suppressed carrier), a comb with N =2 M − m 3 m equally spaced spectral lines, with the same amplitude and phase, can be generated by cascading the modulators and by properly adjusting the applied bias voltage and modulating amplitude, and by appropriately selecting their modulation frequency. To properly adjust the DC bias and modulating RF voltage in each MZM, the expression for the output field from each modulator has to be analyzed. If the DC bias and the RF signal voltages applied to a single modulator are V B and ν s cos(ω s t ), respectively, its normalized output optical field is given by the expression [48] , [56] : where J k is the Bessel function of the first kind and order k , = V B / V π , and α = v s / V π , in which V π is the half-wave voltage of the modulator. Note that according to equation (12), the amplitude of the carrier, first-order sidebands and higher-order sidebands can be adjusted by a proper tuning of the RF-driving voltage α and the DC bias ∈ . The primary objective is to equalize the amplitudes of the carrier and first-order sidebands, and the condition to realize it can be found out from the expression of the output field reduced to these three spectral components: It is important to notice that by using intensity modulators, two degrees of freedom, that is, bias voltage V B and modulating amplitude v s , can be used to equalize the amplitude of the spectral lines having a linear locked-phase difference and to achieve a simultaneous suppression of the higher-order sidebands. This issue makes a significant difference with respect to the use of phase modulators [46] , [47] , [48] , [49] , [50] , [51] where only the modulating voltage can be adjusted, making it impossible to obtain spectral components with the same amplitude and uniform-locked phase. 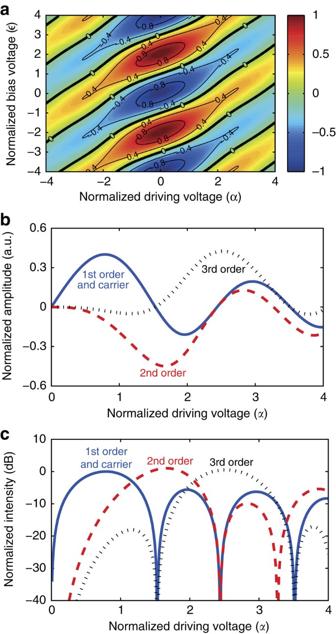Figure 9: Rectangular frequency comb generation with MZMs. (a) Amplitude difference between first-order sidebands and carrier component [−J1(πα/2)sin (π∈/2)−J0(πα/2)cos (π∈/2)]. Equalization of the amplitude between the two first-order sidebands and carrier is only possible if pairs of bias voltage∈and driving voltageαlying over the thick black line at zero level are used. This amplitude equalization not only leads to frequency components with the same power level but also ensures the same phase between them. (b) Field amplitude and (c) power of the three lower-order sidebands as a function of the normalized RF voltage, when the DC bias is set to equalize carrier and first-order sideband amplitudes. Power levels have been normalized to the maximum power reached by the first-order sidebands. Figure 9a shows a contour plot representing the amplitude difference between the first-order sidebands and the carrier (that is, − J 1 ( πα /2)sin( π ∈ /2)− J 0 ( πα /2)cos( π ∈ /2)) as a function of the normalized voltages α and ∈ . The figure indicates that there are many combinations of α and (represented by the thick solid lines at zero level in the contour plot) that equalize the amplitudes of the carrier and the first-order sidebands. Actually, as depicted in Fig. 9a , the relation between the optimum bias voltage V B and the driving RF signal amplitude v s that fulfils this condition is a periodic function, which can be simply obtained from equation (13): Figure 9: Rectangular frequency comb generation with MZMs. ( a ) Amplitude difference between first-order sidebands and carrier component [− J 1 ( πα /2)sin ( π ∈ /2)− J 0 ( πα /2)cos ( π ∈ /2)]. Equalization of the amplitude between the two first-order sidebands and carrier is only possible if pairs of bias voltage ∈ and driving voltage α lying over the thick black line at zero level are used. This amplitude equalization not only leads to frequency components with the same power level but also ensures the same phase between them. ( b ) Field amplitude and ( c ) power of the three lower-order sidebands as a function of the normalized RF voltage, when the DC bias is set to equalize carrier and first-order sideband amplitudes. Power levels have been normalized to the maximum power reached by the first-order sidebands. Full size image Although all valid combinations of V B and v s given by equation (14) and graphed in Fig. 9a provide equalized amplitudes for the three frequency components (two first-order sidebands and carrier), their absolute amplitude can vary considerably. Moreover, phase and amplitude of the higher-order sidebands can also be adjusted by changing the operating bias point and the modulating RF voltage amplitude. Figure 9b shows the amplitude of the three lower-order sidebands as a function of the normalized RF-driving voltage α , when the optimum bias is set according to equation (14). It can be observed that a high amplitude of the first-order sidebands (equal to the carrier amplitude) together with a low amplitude of higher-order sidebands is only possible if the normalized RF voltage α is set to be lower than 0.8. Other voltage conditions result in lower suppression of the higher-order sidebands, leading to a frequency comb with badly equalized frequency components. It must be pointed out that the higher-order sidebands have to be strongly suppressed to confine the sinc-pulse sequence into the Nyquist bandwidth. Figure 9c shows the power level of the three higher-order sidebands in dB scale versus the normalized RF voltage, when the bias point is set at its optimum value according to equation (14) (power levels in the figure have been normalized to the maximum power of the equalized first-order sidebands). The figure points out that, as previously mentioned, strong suppression of the higher-order sidebands can only be achieved by using a low RF signal amplitude. Although only the three lower-order sidebands are analyzed here, higher-order sidebands are expected to have much reduced power levels because of the lower amplitude of the higher-order Bessel functions J k in this driving voltage range. This can be readily justified as a result from the asymptotic form of the Bessel function J k ( x )~ x k for small argument x . According to Fig. 9c , the maximum power of the carrier and the first-order sidebands can be reached using a driving voltage v s =0.8 V π . This condition offers a 15-dB suppression of the second-order sidebands (see red-dashed line in the figure). However, stronger higher-order sideband suppression can be achieved by a slight reduction of the driving voltage, which also leads to a small power reduction of carrier and first-order sidebands. Thus, for instance, using a modulating voltage v s =0.32 V π , a higher-order sideband suppression of more than 30 dB can be achieved with a power reduction of 4.5 dB on the carrier and the first-order sidebands with respect to the maximum reachable power level. Thus, arbitrary out-of-band suppression can be obtained using lower RF voltages, while the power reduction of carrier and first-order sidebands can be easily compensated by optical amplification. To implement the proposed idea, a proof-of-concept set-up is implemented in this paper based on two cascaded MZM, driven by independent RF generators; however, there are many ways to extend and improve the proposed set-up. Instead of a second generator, a frequency tripler and a phase shifter can be used to drive both modulators. In addition, the number of frequency lines generated by each modulator can be increased combining two or even more RF signals in the electrical domain. In this way, the set-up can even be compacted to operate using a single MZM. Further, shorter pulses can be generated with higher bandwidth modulators, or by the exploitation of the second-order sidebands [48] , [56] and the simultaneous suppression of the out-of-phase components. According to equation (12), all odd-order sidebands can be simultaneously suppressed using a bias voltage V B = ∈ V π , ∈ being an even number. Under this condition, only the carrier and even-order sidebands could exit the modulator. While higher-order sidebands are expected to be very low, a strong carrier can still exist. Unfortunately, the carrier component is out-of-phase with respect to the second-order sidebands, and therefore it needs to be conveniently suppressed. This suppression can be achieved with a proper RF-modulating amplitude, so that the Bessel function of zero order in equation (12) vanishes. This optimal condition is given by a driving voltage v s ≈1.52 V π . Figure 9c points out that in such an optimal operating point, the second-order sidebands can be exploited together with a high suppression of the carrier and odd-order sidebands. This would lead to a broader frequency comb and hence to shorter sinc-shaped Nyquist pulses. The main practical limitation for this scheme is given by the possibility that the required driving voltage can exceed the maximum RF power allowed by the MZM, and therefore modulators with reduced V π could be more suitable for this purpose. The proposed technique can produce sinc-shaped Nyquist pulse sequences of very high quality; however, slight deviations from the ideal sinc shape can be expected in the implementation because of some practical limitations, such as the laser linewidth or the chirp induced by the modulators, leading to small phase differences among the comb spectral components. Possible improvements can be obtained using narrower linewidth optical sources, such as Brillouin lasers with linewidth in the Hz range [57] , or employing optimized x-cut chirp-free intensity modulators [58] . How to cite this article: Soto, M. A. et al. Optical sinc-shaped Nyquist pulses of exceptional quality. Nat. Commun. 4:2898 doi: 10.1038/ncomms3898 (2013).